EphrinB2 controls vessel pruning through STAT1-JNK3 signalling Angiogenesis produces primitive vascular networks that need pruning to yield hierarchically organized and functional vessels. Despite the critical importance of vessel pruning to vessel patterning and function, the mechanisms regulating this process are not clear. Here we show that EphrinB2, a well-known player in angiogenesis, is an essential regulator of endothelial cell death and vessel pruning. This regulation depends upon phosphotyrosine-EphrinB2 signalling repressing c-jun N-terminal kinase 3 activity via STAT1. JNK3 activation causes endothelial cell death. In the absence of JNK3, hyaloid vessel physiological pruning is impaired, associated with abnormal persistence of hyaloid vessels, defective retinal vasculature and microphthalmia. This syndrome closely resembles human persistent hyperplastic primary vitreus (PHPV), attributed to failed involution of hyaloid vessels. Our results provide evidence that EphrinB2/STAT1/JNK3 signalling is essential for vessel pruning, and that defects in this pathway may contribute to PHPV. During development and in adult mammals, the vessel network expands through angiogenic sprouting into areas with increased need for nutrients and oxygen, and subsequently undergoes complex remodelling through branch pruning, pericyte coverage and basement membrane deposition to generate a quiescent and mature vasculature [1] . Although considerable progress has been made in clarifying the signals that orchestrate endothelial cell sprouting, less is known about the mechanisms controlling blood vessel pruning despite the critical importance of this process to the patterning, density and function of blood vessels. Capillary involution is evident in the hyaloid vessels, which fully regress after providing a temporary blood supply during eye development [2] , in the primitive retinal vessels, which mature into a stable plexus [3] or degenerate after exposure to hyperoxia [4] , and in the tumour vasculature, where degenerating vessels border dense and chaotic vasculature [1] . Reduced blood flow [5] , [6] , vascular endothelial growth factor (VEGF) reduction [7] , [8] , Dll4/Notch activation [3] , [9] , FYVE expression [10] , exposure to tumour necrosis factor TNFα or interferon (IFN)-γ (refs 11 , 12 ), loss of Nrarp [13] and light-induced responses [14] can provide death signals to the vascular endothelium. EphrinB2, a transmembrane ligand for Eph receptors that is expressed on arterial endothelium, plays pivotal roles in angiogenesis during development and disease [15] , [16] , [17] , [18] . Genetic experiments in mice have shown that the global inactivation of Efnb2 (refs 19 , 20 ), the targeted inactivation of Ephb2 to the endothelium [21] , or replacement of the endogenous gene by complementary DNA encoding a mutant EphrinB2 that lacks 66 amino-acid residues of the cytoplasmic tail [22] similarly impair early embryonic angiogenesis and cause lethality. Since this EphrinB2 cytoplasmic deletion did not impair EphB4 receptor activation, it follows that EphrinB2 intrinsic signalling from the cytoplasmic domain is critical to vascular development [22] , [23] . Mechanistic studies have revealed that EphrinB2 signalling involving PDZ interactions promotes VEGF receptor 2 (VEGFR2) activation and angiogenic sprouting, whereas phosphotyrosine-dependent EphrinB2 signalling does not [24] , [25] . However, EphrinB2 is tyrosine phosphorylated in angiogenic vessels [26] . Genetic evidence has demonstrated that phosphotyrosine-dependent EphrinB2 signalling regulates cell–cell adhesion and cell movement by recruiting Grb4 (ref. 17 ) but has not been linked to post-angiogenic vessel remodelling or pruning. Here we identify a novel pathway controlled by EphrinB2 that is critical for regulation of vessel survival and pruning in the vasculature of the eye. This pathway links phosphotyrosine-dependent EphrinB2 signalling with repression of JNK3 pro-apoptotic activity via STAT1. In the absence of tyrosine-phosphorylated EphrinB2 (p-EphrinB2) or JNK3, physiological involution of hyaloid vessels is impaired producing a syndrome that resembles human persistent hyperplastic primary vitreus (PHPV). EphrinB2 controls vessel pruning in the eye To evaluate the contribution of EphrinB2 phosphotyrosine-dependent signalling to vessel pruning of the ocular vasculature, we analysed knock-in mice with a targeted mutation of the five conserved tyrosine residues ( EphrinB2 5Y/5Y mice) in the cytoplasmic tail, which impairs this signalling [23] . The ocular vasculature comprises the hyaloid and retinal vascular systems [27] . Hyaloid vessels, an arterial vascular network fully developed at birth that supports development of the eye, regress as the retinal vasculature develops [2] . Wild-type (WT) hyaloid vessels broadly express tyrosine-p-EphrinB at postnatal day (p)4, which is expectedly absent from the EphrinB2 5Y/5Y vessels ( Supplementary Fig. 1a ). We found that hyaloid vessels in EphrinB2 5Y/5Y mice display significantly reduced branching compared with EphrinB2 WT/WT mice at p3 and p4, vessel thinning and appearance of gaps compromising vessels integrity ( Fig. 1a,b ). In 3/21 EphrinB2 5Y/5Y mice, the hyaloid vessels were segmentally missing and the eyes were grossly abnormal ( Supplementary Fig. 1b,c ). Type IV collagen immunostaining showed increased regression of hyaloid vessels (collagen IV + CD31 − sleeves) in the EphrinB2 5Y/5Y mice compared with EphrinB2 WT/WT ( Fig. 1c–e ), whereas endothelial cell proliferation in hyaloid vessels (marked by Ki67) was similarly low ( Fig. 1f,g ). The number of red blood cells in the hyaloid vessels was significantly reduced in EphrinB2 5Y/5Y hyaloid vessels compared with control at p3 and p4 ( Fig. 2a–c ). This red cell reduction was attributable to decreased hyaloid vessel perfusion in EphrinB2 5Y/5Y mice compared with EphrinB2 WT/WT ( Fig. 2d–f ). 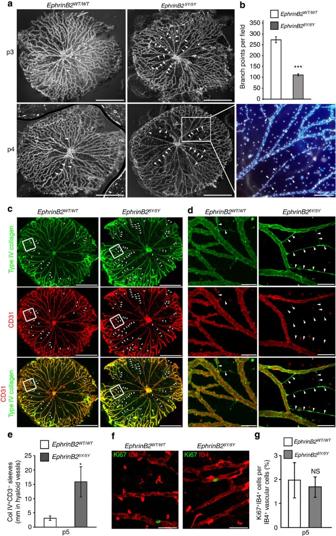Figure 1: Defective hyaloid vessels inEphrinB25Y/5Ymice. (a) Reduced hyaloid vessel branching and thin vessels (arrowheads) in p3 and p4EphrinB25Y/5Ymice compared withEphrinB2WT/WTmice (scale bars, 500 μm). Representative thin/degenerating p4 hyaloid vessels with evidence of gaps are magnified (scale bars, 100 μm). Hyaloid vessels (white) are identified by phase contrast imaging in low magnification panels; DAPI (blue)/phase contrast field imaging identifies vessels in the magnification. (b) Quantification of branching inWTand mutant p4 hyaloid vessels (means±s.d.;n=5 per group). (c,d) Vascular sleeves (type IV collagen+CD31−) are visualized in p5 hyaloid vessels fromEphrinB2WT/WTandEphrinB25Y/5Ymice. Low magnification images (c; scale bars, 500 μm) are magnified (d; scale bars, 50 μm); arrowheads: sleeves. Type IV collagen: green CD31: red. (e) Quantification of vascular sleeves in p5 hyaloid vessels (total length of sleeves in mm; means±s.d.;n=4 per group). (f) Ki67 immunostaining marks proliferating cells in hyaloid vessels stained by IB4; scale bars, 50 μm. Ki67: green; IB4: red. (g) Quantification of proliferating cells in hyaloid vessels of p5 mice (means±s.d.;n=5 per group).Pvalues, two-tailed Studentt-test: NS, not significant; *P<0.05 and ***P<0.001. Error bars=±s.d. Figure 1: Defective hyaloid vessels in EphrinB2 5Y/5Y mice. ( a ) Reduced hyaloid vessel branching and thin vessels (arrowheads) in p3 and p4 EphrinB2 5Y/5Y mice compared with EphrinB2 WT/WT mice (scale bars, 500 μm). Representative thin/degenerating p4 hyaloid vessels with evidence of gaps are magnified (scale bars, 100 μm). Hyaloid vessels (white) are identified by phase contrast imaging in low magnification panels; DAPI (blue)/phase contrast field imaging identifies vessels in the magnification. ( b ) Quantification of branching in WT and mutant p4 hyaloid vessels (means±s.d. ; n =5 per group). ( c , d ) Vascular sleeves (type IV collagen + CD31 − ) are visualized in p5 hyaloid vessels from EphrinB2 WT/WT and EphrinB2 5Y/5Y mice. Low magnification images ( c ; scale bars, 500 μm) are magnified ( d ; scale bars, 50 μm); arrowheads: sleeves. Type IV collagen: green CD31: red. ( e ) Quantification of vascular sleeves in p5 hyaloid vessels (total length of sleeves in mm; means±s.d. ; n =4 per group). ( f ) Ki67 immunostaining marks proliferating cells in hyaloid vessels stained by IB4; scale bars, 50 μm. Ki67: green; IB4: red. ( g ) Quantification of proliferating cells in hyaloid vessels of p5 mice (means±s.d. ; n =5 per group). P values, two-tailed Student t -test: NS, not significant; * P <0.05 and *** P <0.001. Error bars=±s.d. 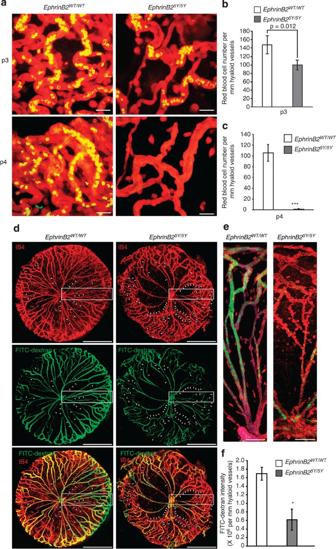Figure 2: Defective perfusion of hyaloid vessels inEphrinB25Y/5Ymice. (a–c) Reduced number of red blood cells in hyaloid vessels fromEphrinB25Y/5Ycompared withEphrinB2WT/WTmice. Vessels are identified with IB4 (red) staining, red blood cells are identified by autofluorescence (yellow;a; scale bars, 20 μm); quantification of red cells at p3 (b; means±s.d.;n=3 per group;Pvalue, two-tailed Studentt-test) and p4 (c; means±s.d.;n=3 per group). (d–f) Systemic inoculation of FITC-dextran (green) shows defective hyaloid vessels perfusion inEphrinB25Y/5Ymice at p5; arrowheads: poorly perfused hyaloid vessels identified by IB4 (red) staining (d; scale bars, 500 μm). Insets are magnified (e; scale bar: 100 μm); (f) quantification of vessel perfusion (means±s.d.;n=3 per group).Pvalues, two-tailed Studentt-test: *P<0.05 and ***P<0.001. Error bars= ±s.d. Full size image Figure 2: Defective perfusion of hyaloid vessels in EphrinB2 5Y/5Y mice. ( a – c ) Reduced number of red blood cells in hyaloid vessels from EphrinB2 5Y/5Y compared with EphrinB2 WT/WT mice. Vessels are identified with IB4 (red) staining, red blood cells are identified by autofluorescence (yellow; a ; scale bars, 20 μm); quantification of red cells at p3 ( b ; means±s.d. ; n =3 per group; P value, two-tailed Student t -test) and p4 ( c ; means±s.d. ; n =3 per group). ( d – f ) Systemic inoculation of FITC-dextran (green) shows defective hyaloid vessels perfusion in EphrinB2 5Y/5Y mice at p5; arrowheads: poorly perfused hyaloid vessels identified by IB4 (red) staining ( d ; scale bars, 500 μm). Insets are magnified ( e ; scale bar: 100 μm); ( f ) quantification of vessel perfusion (means±s.d. ; n =3 per group). P values, two-tailed Student t -test: * P <0.05 and *** P <0.001. Error bars= ±s.d. Full size image Consistent with these results, cleaved caspase-3, a marker of cell death, was more abundant in EphrinB2 5Y/5Y hyaloid vessels compared with control at p4 and marked degenerating vessels ( Fig. 3a–c ). Hyaloid vessel-associated macrophages were similarly represented and viable in EphrinB2 5Y/5Y and EphrinB2 WT/WT mice at p4, even when associated with degenerating hyaloid vessel segments ( Fig. 3b,d and Supplementary Fig. 2a,b ). Pericytes were also similarly represented and viable along EphrinB2 5Y/5Y and EphrinB2 WT/WT hyaloid vessels at p4 and p5 ( Fig. 3e–g ). 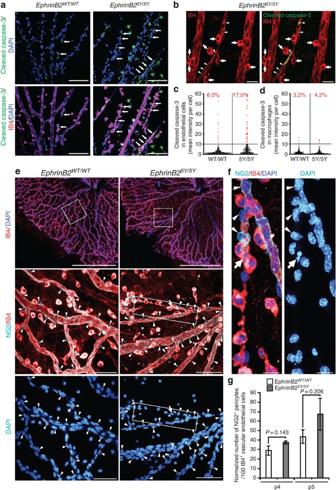Figure 3: Increased cell death in hyaloid vessels ofEphrinB25Y/5Ymice. (a) Cleaved caspase-3 (green) appears more abundant in p4 hyaloid vessels (IB4, pink) fromEphrinB25Y/5Ymice compared withWT; DAPI (blue) identifies cell nuclei; scale bars, 50 μm. Arrows: IB4+cells and cell fragments containing cleaved caspase-3. (b) Hyaloid vessels but not adjacent macrophages are cleaved caspase-3 (green)-positive (arrowheads). IB4 (red) stains hyaloid vessels and macrophages (pointed by arrows, distinct morphology) inEphrinB25Y/5Ymice; scale bars, 20 μm. (c,d) Cleaved caspase-3 is more frequently detected in hyaloid endothelial cells fromEphrinB25Y/5Ycompared withEphrinB2WT/WTmice (c) but not in hyaloid vessel-associated macrophages (d) at p4; in the dot plot, each dot represents 1 cell; horizontal lines denote background immunofluorescence; per cent positive cells are noted. (e) Pericytes (NG2+, cyan) are similarly distributed along hyaloid vessels (stained with IB4, red) ofEphrinB2WT/WTandEphrinB25Y/5Ymice at p4; cell nuclei are identified with DAPI (blue). Arrowheads: pericytes; scale bars, 500 μm (top panels), 50 μm (middle and bottom panels). (f) Inset magnification (scale bars, 10 μm) shows pericytes along a degenerating vessel; arrowheads: pericytes (NG2, cyan); arrow: pyknotic/fragmented endothelial cell nucleus (stained with DAPI, blue); IB4 (red). (g) Pericyte number is measured along hyaloid vessels ofEphrinB2WT/WTandEphrinB25Y/5Ymice at p4 and p5; (means±s.d.;n=3 per group;Pvalues from two-tailed Studentt-test are noted. Error bars= ±s.d.). Figure 3: Increased cell death in hyaloid vessels of EphrinB2 5Y/5Y mice. ( a ) Cleaved caspase-3 (green) appears more abundant in p4 hyaloid vessels (IB4, pink) from EphrinB2 5Y/5Y mice compared with WT ; DAPI (blue) identifies cell nuclei; scale bars, 50 μm. Arrows: IB4 + cells and cell fragments containing cleaved caspase-3. ( b ) Hyaloid vessels but not adjacent macrophages are cleaved caspase-3 (green)-positive (arrowheads). IB4 (red) stains hyaloid vessels and macrophages (pointed by arrows, distinct morphology) in EphrinB2 5Y/5Y mice; scale bars, 20 μm. ( c , d ) Cleaved caspase-3 is more frequently detected in hyaloid endothelial cells from EphrinB2 5Y/5Y compared with EphrinB2 WT/WT mice ( c ) but not in hyaloid vessel-associated macrophages ( d ) at p4; in the dot plot, each dot represents 1 cell; horizontal lines denote background immunofluorescence; per cent positive cells are noted. ( e ) Pericytes (NG2 + , cyan) are similarly distributed along hyaloid vessels (stained with IB4, red) of EphrinB2 WT/WT and EphrinB2 5Y/5Y mice at p4; cell nuclei are identified with DAPI (blue). Arrowheads: pericytes; scale bars, 500 μm (top panels), 50 μm (middle and bottom panels). ( f ) Inset magnification (scale bars, 10 μm) shows pericytes along a degenerating vessel; arrowheads: pericytes (NG2, cyan); arrow: pyknotic/fragmented endothelial cell nucleus (stained with DAPI, blue); IB4 (red). ( g ) Pericyte number is measured along hyaloid vessels of EphrinB2 WT/WT and EphrinB2 5Y/5Y mice at p4 and p5; (means±s.d. ; n =3 per group; P values from two-tailed Student t -test are noted. Error bars= ±s.d.). Full size image Given that hyaloid vessels supply the developing retina, defective hyaloid vessels could impair retinal and eye development. We found that p4 and p5 EphrinB2 5Y/5Y retinas display abnormally reduced vessel branching in the capillary plexus next to the optic nerve ( Fig. 4a,b ), associated with evidence of increased retinal vessel involution at this location ( Fig. 4c,d ). Endothelial cell proliferation was normal in retinal vessels of EphrinB2 5Y/5Y mice both at the sprouting front and in the capillary plexus proximal to the optic nerve ( Fig. 4e,f ). We found that p-EphrinB is broadly detected in retinal vessels of EphrinB2 WT/WT mice at p5, and the absence of p-EphrinB selectively marks vessel segments displaying evidence of degeneration ( Supplementary Fig. 3a ). In addition, we found that adult EphrinB2 5Y/5Y retinas display segmental defects in layer structure involving the centre and middle regions ( Supplementary Fig. 3b ). Together, these results suggested a role of EphrinB2 tyrosine phosphorylation in post-angiogenic regulation of ocular vessels remodelling ( Fig. 4g ). 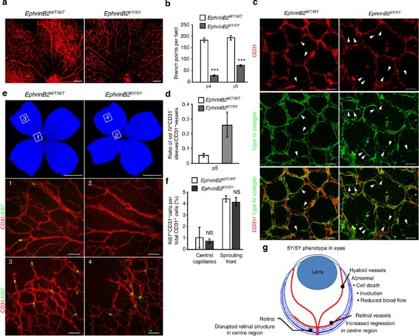Figure 4: Defective retinal vessels inEphrinB25Y/5Ymice. (a) Reduced retinal vessel branching proximal to the optic nerve inEphrinB25Y/5Ymice compared withEphrinB2WT/WTmice at p4; scale bars, 200 μm. Retinal vessels are identified by CD31 (red). (b) Quantification of vessel branching in p4 and p5 retinas proximal to the optic nervein EphrinB25Y/5YandEphrinB2WT/WTmice; mean number±s.d. branch points (n=5 per group). (c,d) Vascular sleeves (type IV collagen+CD31) visualized in retinal vessels at p5 (c; scale bars, 20 μm) are more abundant inEphrinB25Y/5Ycompared withEphrinB2WT/WTmice (d; mean±s.d.,n=5 per group); mean %±s.d. sleeves (n=3 per group); arrowheads: sleeves. Type IV collagen: green; CD31: red. (e,f) CD31+cell proliferation is similar in retinal capillaries ofEphrinB2WT/WTandEphrinB25Y/5Ymice at p5. (e) Proliferation is detected by Ki67 (green) immunostaining in the central retinal capillaries (1,2) and sprouting front (3,4); scale bars, 1 mm (top panels) and 50 μm (middle and bottom panels). CD31 (red) identifies vessels; DAPI (blue) identifies cell nuclei. (f) % Ki67+CD31+cells/total CD31+cells is quantified (mean±s.d.;n=3 per group). (g) Summary representation of ocular defects inEphrinB25Y/5Ymice.Pvalues, two-tailed Studentt-test: NS, not significant; *P<0.05 and ***P<0.001. Error bars: ±s.d. Figure 4: Defective retinal vessels in EphrinB2 5Y/5Y mice. ( a ) Reduced retinal vessel branching proximal to the optic nerve in EphrinB2 5Y/5Y mice compared with EphrinB2 WT/WT mice at p4; scale bars, 200 μm. Retinal vessels are identified by CD31 (red). ( b ) Quantification of vessel branching in p4 and p5 retinas proximal to the optic nerve in EphrinB2 5Y/5Y and EphrinB2 WT/WT mice; mean number±s.d. branch points ( n =5 per group). ( c , d ) Vascular sleeves (type IV collagen + CD31) visualized in retinal vessels at p5 ( c ; scale bars, 20 μm) are more abundant in EphrinB2 5Y/5Y compared with EphrinB2 WT/WT mice ( d ; mean±s.d., n =5 per group); mean %±s.d. sleeves ( n =3 per group); arrowheads: sleeves. Type IV collagen: green; CD31: red. ( e , f ) CD31 + cell proliferation is similar in retinal capillaries of EphrinB2 WT/WT and EphrinB2 5Y/5Y mice at p5. ( e ) Proliferation is detected by Ki67 (green) immunostaining in the central retinal capillaries (1,2) and sprouting front (3,4); scale bars, 1 mm (top panels) and 50 μm (middle and bottom panels). CD31 (red) identifies vessels; DAPI (blue) identifies cell nuclei. ( f ) % Ki67 + CD31 + cells/total CD31 + cells is quantified (mean±s.d. ; n =3 per group). ( g ) Summary representation of ocular defects in EphrinB2 5Y/5Y mice. P values, two-tailed Student t -test: NS, not significant; * P <0.05 and *** P <0.001. Error bars: ±s.d. Full size image EphrinB2 supports endothelial cell survival To examine whether EphrinB2 regulates post-angiogenic vessel pruning by acting directly on endothelial cell survival, we used lentiviral vectors for silencing EphrinB2 (eB2-short hairpin RNAs (shRNAs) nos. 1–4; Supplementary Fig. 4a ) and for expression of WT (eB2-WT) or the phosphotyrosine-deficient (eB2-5Y) EphrinB2. Previously, we showed that eB2-5Y EphrinB2 inhibits phosphorylation of endogenous EphrinB2 in endothelial cells through a dominant-negative effect [26] . We now find that silencing EphrinB2 and expression of eB2-5Y causes significant decrease in HUVECs (human umbilical vein endothelial cells) and HDMECs (human dermal microvascular endothelial cells) viability ( Fig. 5a and Supplementary Fig. 4b,c ). Consistent with this, HUVEC were growth impaired and displayed increased cleavage of poly (ADP-ribose) polymerase, a marker of apoptosis [28] , after EphrinB2 was silenced (eB2-shRNA) or eB2-5Y was expressed ( Fig. 5b,c ). 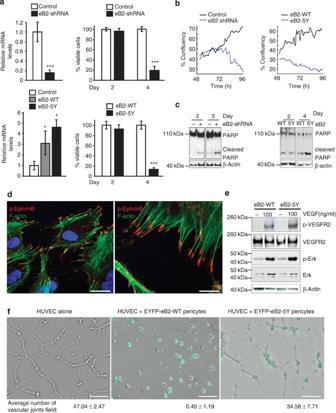Figure 5: EphrinB2 silencing or expression of phosphotyrosine-mutant EphrinB2 promotes endothelial cell death. (a) Viable HUVECs were quantified by flow cytometry on days 2 and 4 post infection with lentivirus control, eB2-shRNA, eB2-WT or eB2-5Y. Effects of silencing are measured by relative mRNA levels (left panels); viability (right panels) is expressed as % of control/eB2-WT (means±s.d.; 3–5 experiments, each performed in triplicate).Pvalues from two-tailed Studentt-test: *P<0.05, ***P<0.001; error bars: ±s.d. (b,c) Growth curves (b) and cleaved poly (ADP-ribose) polymerase detection (c) in HUVEC infected with control, eB2-shRNA, eB2-WT or eB2-5Y. (d) Detection of p-EphrinB (red) in HUVEC from culture. Filamentous (F) actin staining (green) detects stress fibres; DAPI (blue) identifies cell nuclei; scale bars, 20 μm (left panel) and 5 μm (right panel). (e) Levels of p-VEGFR2 (Tyr1175), VEGFR2 and p-ERK (Thr202/Tyr204) are similarly modulated by VEGF in HUVEC transduced with eB2-WT or eB2-5Y. (f) Mesenchymal cells/pericytes expressing EYFP-eB2-5Y (green) are defective at promoting involution of HUVEC vascular structures compared with control pericytes (EYFP-eB2-WT transduced); representative experiment of three; scale bars, 50 μm.The integrity of vascular structures is measured by the average number of joints (mean±s.d.;n=3 experiments per group). Figure 5: EphrinB2 silencing or expression of phosphotyrosine-mutant EphrinB2 promotes endothelial cell death. ( a ) Viable HUVECs were quantified by flow cytometry on days 2 and 4 post infection with lentivirus control, eB2-shRNA, eB2-WT or eB2-5Y. Effects of silencing are measured by relative mRNA levels (left panels); viability (right panels) is expressed as % of control/eB2-WT (means±s.d. ; 3–5 experiments, each performed in triplicate). P values from two-tailed Student t -test: * P <0.05, *** P <0.001; error bars: ±s.d. ( b , c ) Growth curves ( b ) and cleaved poly (ADP-ribose) polymerase detection ( c ) in HUVEC infected with control, eB2-shRNA, eB2-WT or eB2-5Y. ( d ) Detection of p-EphrinB (red) in HUVEC from culture. Filamentous (F) actin staining (green) detects stress fibres; DAPI (blue) identifies cell nuclei; scale bars, 20 μm (left panel) and 5 μm (right panel). ( e ) Levels of p-VEGFR2 (Tyr1175), VEGFR2 and p-ERK (Thr202/Tyr204) are similarly modulated by VEGF in HUVEC transduced with eB2-WT or eB2-5Y. ( f ) Mesenchymal cells/pericytes expressing EYFP-eB2-5Y (green) are defective at promoting involution of HUVEC vascular structures compared with control pericytes (EYFP-eB2-WT transduced); representative experiment of three; scale bars, 50 μm.The integrity of vascular structures is measured by the average number of joints (mean±s.d. ; n =3 experiments per group). Full size image These results together with the observation that EphrinB is phosphorylated in cultured HUVEC ( Fig. 5d and Supplementary Fig. 3c ) indicate that p-EphrinB2 sustains endothelial cell survival. Exogenous FGF2 (fibroblast growth factor-2) and VEGF-A did not prevent HUVEC death after EphrinB2 silencing or expression of eB2-5Y ( Supplementary Table 1 ). Since PDZ-dependent EphrinB2 signalling regulates VEGFR2 activity [24] , we tested whether defective VEGFR2 function accounted for the failure of VEGF to rescue endothelial cells from death. VEGF similarly stimulated VEGFR2 signalling in control and eB2-5Y-expressing endothelial cells ( Fig. 5e ). Thus, cell death induced by the phosphotyrosine-deficient EphrinB2 is not attributable to defective VEGFR2 function. The profound pro-apoptotic effect of eB2-5Y expression in endothelial cells contrasts with the relatively mild vascular phenotype in the EphrinB2 5Y/5Y mice. Since mitigating functions outside the endothelium could contribute to this difference, we focused on pericytes, which promote destabilization/regression of remodelling vessels [26] , [29] . We find that eB2-5Y-mesenchymal cells/pericytes are defective at promoting regression of vascular structures, supporting the integrity of HUVEC-derived vascular structures longer than eB2-WT pericytes ( Fig. 5f ). Given that pericytes appear normally represented along hyaloid vessels of EphrinB2 5Y/5Y mice ( Fig. 3e–g ), the mutant pericytes may serve a similar pro-survival function in the globally deficient EphrinB2 5Y/5Y mice, mitigating the profound pro-apoptotic effect of eB2-5Y expression in endothelial cells. EphrinB2 promotes endothelial cell survival To identify the mechanisms underlying EphrinB2 regulation of endothelial cell survival, we focused on STAT1 and STAT3 since p-EphrinB1 and p-EphrinB2 activate JAK2 (Janus kinase 2)/STAT3 signalling [26] , [30] , [31] , and EphrinB1 associates with STAT1 (ref. 30 ). We found that the proportion of p-STAT1 + (Tyr701) cells was higher in EphrinB2-silenced and EphrinB2-5Y-transduced HUVEC compared with controls, whereas the proportion of p-STAT3 + (Tyr705) cells was similar ( Fig. 6a,b and Supplementary Fig. 5a ). p-STAT1 was mostly nuclear in HUVEC transduced with EphrinB2-5Y consistent with transcriptional activity ( Fig. 6c ). 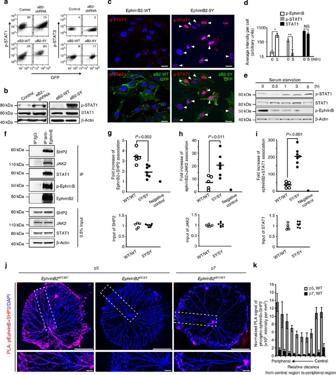Figure 6: EphrinB2 associates with SHP2, JAK2 and STAT1, and modulates STAT1 activity. (a,b) HUVEC infected with eB2-shRNA or eB2-5Y express higher levels of p-STAT1 compared with controls; p-STAT3 levels are similar. Flow cytometry (a; % positive cells is noted on each quadrant; representative of five experiments), immunoblotting (b). (c) Nuclear localization of p-STAT1 (red, arrowheads) in HUVEC transduced with eB2-5Y (GFP: green); little p-STAT1 (red) is detected in HUVEC transduced with eB2-WT (GFP: green); representative images. Scale bars, 20 μm (d) EphB4-Fc activates endogenous p-EphrinB and reduces p-STAT1 levels; quantification (average fluorescence intensity per cell). Results reflect the means±s.d. from three experiments;Pvalues from two-tailed Studentt-test: NS, not significant, *P<0.05, **P<0.01 .Error bars: ±s.d. (e) Serum starvation time-dependently reduces p-EphrinB levels and increases p-STAT1 levels in HUVEC. (f) EphrinB2 associates with SHP2, JAK2 and STAT1 in HUVEC; cell lysates of HUVEC were immunoprecipitated with antibodies to EphrinB2 or control IgG; precipitates and cell lysates were immunoblotted as indicated. (g–i) Quantitative analysis of EphrinB2 association with SHP2, JAK2 and STAT1 in p5 hyaloid vessels fromEphrinB2WT/WT(n=5) andEphrinB25Y/5Y(n=7) mice detected by PEA (top panels). Negative control: reagents alone, no cell lysate. SHP2, JAK2 and STAT1 abundance in PEA input samples (bottom). (j) PLA shows that p-EphrinB associates with SHP2 in hyaloid vessels fromEphrinB2WT/WTmice but not fromEphrinB25Y/5Ymice. Red: EphrinB2+SHP2; blue: DAPI. Dotted line limits amplified areas in lower panels. Scale bars, 500 μm (top panels), 100 μm (bottom panels). (k) Quantification of p-EphrinB+SHP2 proximity co-localization in WT hyaloid vessels regions at p5 and p7. Results (mean±s.d. fluorescence intensity per mm2area) are normalized with DAPI. Error bars=±s.d. Figure 6: EphrinB2 associates with SHP2, JAK2 and STAT1, and modulates STAT1 activity. ( a , b ) HUVEC infected with eB2-shRNA or eB2-5Y express higher levels of p-STAT1 compared with controls; p-STAT3 levels are similar. Flow cytometry ( a ; % positive cells is noted on each quadrant; representative of five experiments), immunoblotting ( b ). ( c ) Nuclear localization of p-STAT1 (red, arrowheads) in HUVEC transduced with eB2-5Y (GFP: green); little p-STAT1 (red) is detected in HUVEC transduced with eB2-WT (GFP: green); representative images. Scale bars, 20 μm ( d ) EphB4-Fc activates endogenous p-EphrinB and reduces p-STAT1 levels; quantification (average fluorescence intensity per cell). Results reflect the means±s.d. from three experiments; P values from two-tailed Student t -test: NS, not significant, * P <0.05, ** P <0.01 .Error bars: ±s.d. ( e ) Serum starvation time-dependently reduces p-EphrinB levels and increases p-STAT1 levels in HUVEC. ( f ) EphrinB2 associates with SHP2, JAK2 and STAT1 in HUVEC; cell lysates of HUVEC were immunoprecipitated with antibodies to EphrinB2 or control IgG; precipitates and cell lysates were immunoblotted as indicated. ( g – i ) Quantitative analysis of EphrinB2 association with SHP2, JAK2 and STAT1 in p5 hyaloid vessels from EphrinB2 WT/WT ( n =5) and EphrinB2 5Y/5Y ( n =7) mice detected by PEA (top panels). Negative control: reagents alone, no cell lysate. SHP2, JAK2 and STAT1 abundance in PEA input samples (bottom). ( j ) PLA shows that p-EphrinB associates with SHP2 in hyaloid vessels from EphrinB2 WT/WT mice but not from EphrinB2 5Y/5Y mice. Red: EphrinB2+SHP2; blue: DAPI. Dotted line limits amplified areas in lower panels. Scale bars, 500 μm (top panels), 100 μm (bottom panels). ( k ) Quantification of p-EphrinB+SHP2 proximity co-localization in WT hyaloid vessels regions at p5 and p7. Results (mean±s.d. fluorescence intensity per mm 2 area) are normalized with DAPI. Error bars=±s.d. Full size image These results suggested that tyrosine p-EphrinB2 represses STAT1 activity in HUVEC. To test this possibility, we examined STAT1 phosphorylation after we induced EphrinB phosphorylation or dephosphorylation. Receptor (EphB4-Fc)-induced activation enhanced EphrinB phosphorylation and reduced ‘constitutive’ p-STAT1 in HUVEC ( Fig. 6d ). Conversely, serum starvation reduced EphrinB phosphorylation and increased p-STAT1 levels in HUVEC ( Fig. 6e ). To identify how p-EphrinB reduces STAT1 activity, we considered SHP2 (SRC homology 2-domain-containing Protein-Tyrosine Phosphatases (PTP)) phosphatase, which dephosphorylates STAT1 (ref. 32 ). EphrinB2 immunoprecipitates from lysates of non-transduced HUVEC contained SHP2 ( Fig. 6f ). They also contained JAK2, a tyrosine kinase that phosphorylates STAT3 (ref. 33 ) and STAT1. This demonstrated the association of endogenous EphrinB2 with SHP2, JAK2 and STAT1. Proximity extension assay (PEA) revealed that EphrinB2 associates with SHP2 in hyaloid vessels from EphrinB2 WT/WT mice, but to a significantly lower degree in hyaloid vessels from EphrinB2 5Y/5Y littermates ( Fig. 6g ). PEA also confirmed the physiological association of EphrinB2 with JAK2 and STAT1 in vivo , and showed that EphrinB2-5Y associates with JAK2 and STAT1 more than WT EphrinB2 ( Fig. 6h,i ). Proximity ligation assay (PLA) imaging further showed that p-EphrinB and SHP2 are specifically associated in hyaloid vessels from EphrinB2 WT/WT ( Fig. 6j ). Based on these results, we examined whether the degree of association between p-EphrinB and SHP2 changes during physiological involution of hyaloid vessels. We found that concurrent with a decline in the proportion of hyaloid p-EphrinB + cells (39.9% at p5 AND 20.8% at p7), p-EphrinB/SHP2 interaction also declines in WT hyaloid vessels from p5 to p7 ( Fig. 6k ). Most hyaloid vessel involution proceeds in regions intermediate between the centre and the periphery at p4–p7 ( Supplementary Fig. 5b,c ). Consistent with this, most p-EphrinB/SHP2 interaction localizes in the peripheral and central regions of hyaloid vessels at p5/p7, where most p-EphrinB + cells reside ( Fig. 6j,k AND Supplementary Fig. 5b,c ). Together, these results suggest that p-EphrinB2 sustains endothelial cell viability by recruiting SHP2, which inactivates STAT1. Consistent with this, SHP2 silencing increased p-STAT1 levels in HUVEC ( Supplementary Fig. 6a ). In addition, STAT1 silencing ( Supplementary Fig. 6b ) increased HUVEC viability compromised by expression of EphrinB2-5Y ( Fig. 7a ). 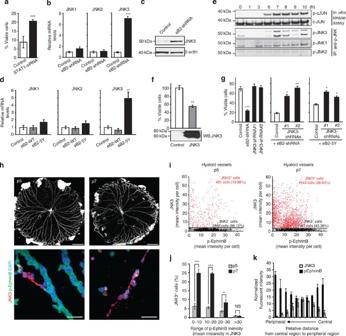Figure 7: JNK3 is expressed in regressing hyaloid vessels and mediates EphrinB2-dependent endothelial cell death. (a) STAT1 silencing augments cell viability in HUVEC expressing eB2-5Y. Results reflect the means±s.d. from three experiments; error bars: ±s.d. (b,c) eB2-shRNA augments JNK3 mRNA (b; means±s.d. from three experiments; error bars: ±s.d.) and protein (c) expression in HUVEC. (d) Transduction of eB2-5Y but not eB2-WT augments JNK3 expression in HUVEC; means±s.d. from three experiments; error bars: ±s.d. (e) Time-dependent JNK3 and cJUN activation in serum-starved HUVEC. Cell lysates from serum-starved HUVEC were tested at the indicated time points for kinase activity and content of p-JNK1, p-JNK2 and p-JNK3 after IP with anti-p-JNK antibody. (f) JNK3 transduction reduces HUVEC viability; means±s.d. from 3 experiments; error bars: ±s.d. (g) JNK3 silencing improves HUVEC viability compromised by eB2-shRNA and B2-5Y transduction; means±s.d. from 3–5 experiments; error bars: ±s.d. (h) JNK3 is detected in p5 and p7WThyaloid vessels. Degenerating hyaloid vessels are marked by anti-JNK3 antibody staining (red); p-EphrinB immunostaining (green) is absent from JNK3+ hyaloid vessels; DAPI (blue). Scale bars, 200 μm (top panels) and 50 μm (bottom panels). (i–k) Immunostaining reveals an inverse relationship between JNK3 and p-EphrinB fluorescence intensity in individual IB4+cells within p5 and p7WThyaloid vessels. Cell distribution based on JNK3 and p-EphrinB mean fluorescence intensity; each dot represents one cell (i); the bar graphs show (j) the means (n=100–300 per group) and range (±s.d. error bars) of p-EphrinB fluorescence intensity in JNK3+cells and (k) the geographical distribution within hyaloid vessels of JNK3+(mean fluorescence intensity ≥3.5)/p-EphrinB+(mean fluorescence intensity ≥30) cells (means±s.d.;n=4 areas per group); fluorescence intensity values in each region are normalized by DAPI.Pvalues from two-tailed Studentt-test: NS, not significant; *P<0.05, **P<0.01 and ***P<0.001. Figure 7: JNK3 is expressed in regressing hyaloid vessels and mediates EphrinB2-dependent endothelial cell death. ( a ) STAT1 silencing augments cell viability in HUVEC expressing eB2-5Y. Results reflect the means±s.d. from three experiments; error bars: ±s.d. ( b , c ) eB2-shRNA augments JNK3 mRNA ( b ; means±s.d. from three experiments; error bars: ±s.d.) and protein ( c ) expression in HUVEC. ( d ) Transduction of eB2-5Y but not eB2-WT augments JNK3 expression in HUVEC; means±s.d. from three experiments; error bars: ±s.d. ( e ) Time-dependent JNK3 and cJUN activation in serum-starved HUVEC. Cell lysates from serum-starved HUVEC were tested at the indicated time points for kinase activity and content of p-JNK1, p-JNK2 and p-JNK3 after IP with anti-p-JNK antibody. ( f ) JNK3 transduction reduces HUVEC viability; means±s.d. from 3 experiments; error bars: ±s.d. ( g ) JNK3 silencing improves HUVEC viability compromised by eB2-shRNA and B2-5Y transduction; means±s.d. from 3–5 experiments; error bars: ±s.d. ( h ) JNK3 is detected in p5 and p7 WT hyaloid vessels. Degenerating hyaloid vessels are marked by anti-JNK3 antibody staining (red); p-EphrinB immunostaining (green) is absent from JNK 3 + hyaloid vessels; DAPI (blue). Scale bars, 200 μm (top panels) and 50 μm (bottom panels). ( i – k ) Immunostaining reveals an inverse relationship between JNK3 and p-EphrinB fluorescence intensity in individual IB4 + cells within p5 and p7 WT hyaloid vessels. Cell distribution based on JNK3 and p-EphrinB mean fluorescence intensity; each dot represents one cell ( i ); the bar graphs show ( j ) the means ( n =100–300 per group) and range (±s.d. error bars) of p-EphrinB fluorescence intensity in JNK3 + cells and ( k ) the geographical distribution within hyaloid vessels of JNK3 + (mean fluorescence intensity ≥3.5)/p-EphrinB + (mean fluorescence intensity ≥30) cells (means±s.d. ; n =4 areas per group); fluorescence intensity values in each region are normalized by DAPI. P values from two-tailed Student t -test: NS, not significant; * P <0.05, ** P <0.01 and *** P <0.001. Full size image JNK3 mediates cell death induced by EphrinB2 dephosphorylation To investigate the mechanisms underlying EphrinB2/STAT1-induced cell death, we hypothesized an effector role for MAPK10/JNK3, a kinase whose activation is linked to cell death [34] . IFNγ, an inducer of p-STAT1 and endothelial cell death [12] , promotes MAPK10/JNK3 expression in HUVEC, but not the expression of MAPK8/JNK1 or MAPK9/JNK2 ( http://sbmdb.genome.rcast.u-tokyo.ac.jp/huvecdb/main_search.jsp ; JNK3: probes 237413_at, JNK1: 226046_at and JNK2: 203218_at HUVEC database). Also, the promoter region of JNK3 contains a putative binding site for STAT1 (Champion Chip transcription factor Search portal, DECODE database, SABiosciences). EphrinB2 silencing increased JNK3 expression in HUVEC, but not the expression of JNK1 and JNK2 ( Fig. 7b,c ). Transduced EphrinB2-5Y induced greater expression of JNK3 than EphrinB2WT, but minimally changed JNK1 and JNK2 expression in HUVEC ( Fig. 7d ). Immunoprecipitation (IP)/immunoblotting further revealed that endogenous JNK3 is time-dependently phosphorylated in serum-starved HUVEC under conditions that lead to EphrinB2 dephosphorylation, whereas JNK1 or JNK2 are not phosphorylated ( Fig. 7e ). In vitro kinase assays further showed that endogenous p-JNK3 induced in HUVEC by serum starvation is biologically active as assessed by phosphorylation of the exogenous target, cJUN ( Fig. 7e ). Functionally, forced expression of JNK3 promoted HUVEC death ( Fig. 7f ), and the silencing of JNK3 increased HUVEC viability after EphrinB2 silencing or expression of EphrinB2-5Y ( Fig. 7g and Supplementary Fig. 6c ). This indicated that the pro-survival function of EphrinB2 in this system is linked to JNK3 repression. Next we examined whether JNK3 plays a role in the physiological involution of hyaloid vessels. We detected JNK3 in p5 and p7 hyaloid vessels, particularly at sites of vessel degeneration where p-EphrinB is not detected ( Fig. 7h and Supplementary Fig. 6d ). By measuring JNK3 and p-EphrinB staining intensities in individual cells within hyaloid vessels, we found a time-dependent (from p5 to p7) increase of IB4 + /JNK3 + cells (13.9–56.6%) and a decrease of IB4 + /p-EphrinB + cells (39.9–20.8%; Fig. 7i,j ). JNK3 high cells generally showed no or low levels of p-EphrinB2 signals ( Fig. 7j ), and clustered at a mid relative distance between the centre and the periphery of hyaloid vessels, where most vessel degeneration occurs at p4–p7 ( Fig. 7k and Supplementary Fig. 5b,c ). The p-EphrinB high /JNK3 low cells clustered in the more viable peripheral and central regions of hyaloid vessels ( Fig. 7k ). Thus, JNK3 marks endothelial cell death in physiologically involuting hyaloid vessels as they lose EphrinB phosphorylation. We further examined whether p-STAT1 binds to the JNK3 promoter as predicted in silico . Chromatin IP in lysates of HUVEC expressing endogenous p-STAT1 after serum starvation ( Fig. 6e ) showed that p-STAT1 binds to the JNK3 promoter region predicted to bind p-STAT1 ( Fig. 8a ). Maximal p-STAT1/JNK3 promoter interaction temporally coincided with maximal p-STAT1 activation and was similar in magnitude to that found in IFNγ-stimulated HUVEC ( Fig. 8a ). In a reporter assay, WT EphrinB2 significantly reduced JNK3 promoter activity driven by the transfected JAK2 (but not dominant-negative JAK2) plus STAT1, whereas EphrinB2-5Y exerted an insignificant repressive effect ( Fig. 8b ). 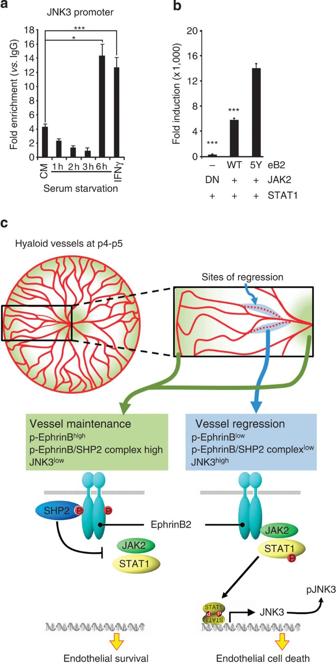Figure 8: JNK3 is a target of p-STAT1 regulation. (a) HUVEC-endogenous p-STAT1 induced by serum starvation or IFNγ (10 ng ml−1) stimulation specifically binds to JNK3 promoter region. Chromatin IP with p-STAT1 antibodies or control IgG; precipitated DNA was measured by quantitative PCR with specific primers for JNK3 promoters. CM: HUVEC complete medium. Results show means (±s.d. shown as error bars) from five replicates.Pvalues from two-tailed Studentt-test: *P<0.05 and ***P<0.001. (b) WT EphrinB2 represses JAK2+STAT1-driven JNK3 promoter activity; GLuc dual-reporter assay; means (±s.d. shown as error bars) of five experiments.Pvalues from two-tailed Studentt-test: ***P<0.001. The JNK3 reporter plasmid was co-transfected in HEK293T cells with expression plasmids for JAK2+STAT1; dominant-negative (DN) JAK2+STAT1; JAK2+STAT1+eB2-WT or JAK2+STAT1+eB2-5Y. (c) Schematic representation of experimental results. Figure 8: JNK3 is a target of p-STAT1 regulation. ( a ) HUVEC-endogenous p-STAT1 induced by serum starvation or IFNγ (10 ng ml −1 ) stimulation specifically binds to JNK3 promoter region. Chromatin IP with p-STAT1 antibodies or control IgG; precipitated DNA was measured by quantitative PCR with specific primers for JNK3 promoters. CM: HUVEC complete medium. Results show means (±s.d. shown as error bars) from five replicates. P values from two-tailed Student t -test: * P <0.05 and *** P <0.001. ( b ) WT EphrinB2 represses JAK2+STAT1-driven JNK3 promoter activity; GLuc dual-reporter assay; means (±s.d. shown as error bars) of five experiments. P values from two-tailed Student t -test: *** P <0.001. The JNK3 reporter plasmid was co-transfected in HEK293T cells with expression plasmids for JAK2+STAT1; dominant-negative (DN) JAK2+STAT1; JAK2+STAT1+eB2-WT or JAK2+STAT1+eB2-5Y. ( c ) Schematic representation of experimental results. Full size image These results support a model ( Fig. 8c ) in which hyaloid vessel regression proceeds principally in regions intermediate between the central and peripheral regions at p4–p5. At this time, hyaloid vessels in the peripheral and central regions do not regress. Non-regressing hyaloid vessels show high-level p-EphrinB. This p-EphrinB provides prosurvival signals by associating with the phosphatase SHP2, which dephosphorylates STAT1; proapoptotic JNK3 is not active. Instead, regressing hyaloid vessels show low-level p-EphrinB, resulting in increased cell death. Non phosphorylated EphrinB is poorly associated with SHP2; JNK3 is induced and is active. In sum, EphrinB2/JNK3 signalling emerges as a key regulator of endothelial cell survival and post-angiogenic vessel remodelling. JNK3 regulates involution of hyaloid and retinal vessels A prediction from this model is that JNK3 deficiency reduces physiological involution of hyaloid vessels. Analysis of JNK3 −/− mice at p5 found that 77% of mice (10/13 mice) from eight litters showed an abnormal eye phenotype, which affected both eyes in 30% of mice (3/10) and one eye in 70% of mice (7/10). In the seven most severe cases, the eye and lens were significantly smaller than controls, and the retina visualized from the rear presented irregular folds/pockets that were not found in the controls ( Fig. 9a,b and Supplementary Fig. 7a,b ). The space separating the retina from the lens, which normally contains the vitreous elements, was reduced in size in these JNK3 −/− mice, as it was occupied by a retrolental mass, mostly staining with IB4 ( Fig. 9c ). p-EphrinB marked viable-appearing IB4 + cells lining the posterior aspect of the lens (arrowheads) in the control and in the JNK3 −/− mice ( Fig. 9d ). The absence of p-EphrinB in IB4 + cells (arrows) coincided with morphological evidence of cell degeneration in the controls, but no such evidence of degeneration was noted in the JNK3 −/− IB4 + cells ( Fig. 9d ). Histologically, the JNK3 −/− retrolental mass appears as an abnormal vascular-type structure, mostly composed of IB4 + cells mixed with NG2 + pericytes, and infiltrated with F4/80 + macrophages ( Fig. 9e ). This mass is absent from JNK3 +/+ eyes, showing instead normal-appearing IB4 + hyaloid vessels associated with NG2 + and F4/80 + cells ( Fig. 9e ). The JNK3 −/− retrolental mass (arrows) did not stain for cleaved caspase-3, which was detected in a proportion of control hyaloid cells (arrowheads), presumably physiologically degenerating ( Fig. 9f ). The superficial retinal vasculature, normally present at p5 extending outwards from the optic nerve, was less extensive in JNK3 −/− retinas ( Supplementary Fig. 7c,d ). Instead, clusters of JNK3 −/− hyaloid vessels appeared to form a substitute retinal vasculature, as there was evidence of angiogenic sprouting and filopodia formation at the edge of the JNK3 −/− hyaloid vascular plexus with penetration of the hyaloid vessels into the retinal layer ( Supplementary Fig. 7e–g ). In the three less severe cases, the hyaloid vessels displayed significantly greater branching compared with controls at p5 consistent with reduced involution, and the JNK3 −/− eyes were abnormally small. In addition, 36% of adult (11–16 weeks old, n =11) JNK3 −/− mice displayed a pathological retrolental mass, consistent with an abnormal persistence of hyaloid vessels ( Fig. 9g,h ). Thus, JNK3 deficiency causes abnormal persistence of hyaloid vessels and ocular pathology in mice. 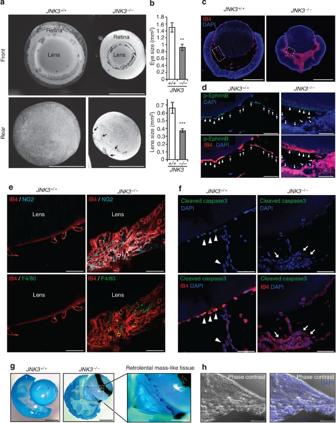Figure 9: Phenotypes ofJNK3−/−eyes. (a)JNK3−/−mice display microphthalmia and abnormal retinal folding. Front and rear view of p5 eyes fromJNK3+/+andJNK3−/−mice. Arrows: abnormal retinal folds and pockets. Scale bars, 1 mm. (b) Measurements of eye and lens size in eye sections ofJNK3+/+andJNK3−/−p5 mice. The results reflect the means ±s.d.;n=3 mice per group;Pvalues from two-tailed Studentt-test: **P<0.01 and ***P<0.001. (c) Presence of an abnormal retrolental mass in the vitreous region ofJNK3−/−mice. IB4 staining of eye sections in representative p5JNK3+/+andJNK3−/−pups; scale bars, 500 μm. IB4: red; DAPI: blue. Insets are enlarged ind. (d) The retrolental mass inJNK3−/−mice is stained with IB4 (red), p-EphrinB (green) and DAPI (blue). Arrowheads: p-EphrinB+/IB4+cells; arrows: p-EphrinB−/IB4+cells; scale bars, 50 μm. (e) Retrolental mass from aJNK3−/−mouse at p5 contains NG2+pericytes (cyan) and F4/80+macrophages (green) within an IB4+vascular-type structure (red). A littermateJNK+/+mouse displays no retrolental mass; hyaloid vessels are located on the lens. Images are from sections of the entire eyeball. Scale bars, 50 μm. (f) The retrolental mass ofJNK3−/−mice is cleaved caspase-3-negative. Cleaved caspase-3: green; IB4: red; DAPI: blue. Arrowheads: cleaved caspase-3+/IB4+cells; arrows: cleaved caspase-3−/IB4+retrolental mass. Scale bars, 50 μm. (g) A pathological retrolental mass is detected in the eye of a 16-week-oldJNK3−/−mouse but not in aJNK3+/+littermate (scale bars: 1 mm); inset is magnified on the right (scale bar: 500 μm); tissues were stained with colloidal Coomassie G-250. (h) Phase contrast imaging of the unstained or DAPI-stained (blue) retrolental mass shown ing; scale bars, 100 μm. Figure 9: Phenotypes of JNK3 −/− eyes. ( a ) JNK3 −/− mice display microphthalmia and abnormal retinal folding. Front and rear view of p5 eyes from JNK3 +/+ and JNK3 −/− mice. Arrows: abnormal retinal folds and pockets. Scale bars, 1 mm. ( b ) Measurements of eye and lens size in eye sections of JNK3 +/+ and JNK3 −/− p5 mice. The results reflect the means ±s.d. ; n =3 mice per group; P values from two-tailed Student t -test: ** P <0.01 and *** P <0.001. ( c ) Presence of an abnormal retrolental mass in the vitreous region of JNK3 −/− mice. IB4 staining of eye sections in representative p5 JNK3 +/+ and JNK3 −/− pups; scale bars, 500 μm. IB4: red; DAPI: blue. Insets are enlarged in d . ( d ) The retrolental mass in JNK3 −/− mice is stained with IB4 (red), p-EphrinB (green) and DAPI (blue). Arrowheads: p-EphrinB + /IB4 + cells; arrows: p-EphrinB − /IB4 + cells; scale bars, 50 μm. ( e ) Retrolental mass from a JNK3 −/− mouse at p5 contains NG2 + pericytes (cyan) and F4/80 + macrophages (green) within an IB4 + vascular-type structure (red). A littermate JNK +/+ mouse displays no retrolental mass; hyaloid vessels are located on the lens. Images are from sections of the entire eyeball. Scale bars, 50 μm. ( f ) The retrolental mass of JNK3 −/− mice is cleaved caspase-3-negative. Cleaved caspase-3: green; IB4: red; DAPI: blue. Arrowheads: cleaved caspase-3 + /IB4 + cells; arrows: cleaved caspase-3 − /IB4 + retrolental mass. Scale bars, 50 μm. ( g ) A pathological retrolental mass is detected in the eye of a 16-week-old JNK3 −/− mouse but not in a JNK3 +/+ littermate (scale bars: 1 mm); inset is magnified on the right (scale bar: 500 μm); tissues were stained with colloidal Coomassie G-250. ( h ) Phase contrast imaging of the unstained or DAPI-stained (blue) retrolental mass shown in g ; scale bars, 100 μm. Full size image p-EphrinB in PHPV The abnormal persistence of fetal hyaloid vasculature in humans is associated with a syndrome known as ‘PHPV’, which includes microphthalmia and leukocoria [35] , [36] . In humans, hyaloid vessels involute before birth. Consistent with previous descriptions, we find that PHPV eyes (six examined) display an abnormal retrolental fibrovascular mass, which physically interacts with the neuro-retina causing tractional retinal detachment and degeneration ( Fig. 10a ). Human CD31 immunostaining revealed endothelial cells co-expressing p-EphrinB in a PHPV retrolental mass; JNK3 was not detected ( Fig. 10b and Supplementary Fig. 8a–c ). By PLA, p-EphrinB was specifically associated with SHP2 in retrolental CD31 + cells ( Fig. 10c and Supplementary Fig. 8d,e ). Also, EphrinB2 was specifically associated with STAT1 ( Fig. 10d and Supplementary Fig. 8d,e ), but minimally with p-STAT1 ( Fig. 10e and Supplementary Fig. 8d,e ) in retrolental CD31 + cells. Since we showed that p-EphrinB/SHP2 sustain endothelial cell viability preventing physiological involution of hyaloid vessels, the detection of p-EphrinB/SHP2 in the retrolental mass of PHPV is consistent with a pathogenetic role of p-EphrinB in the abnormal persistence of hyaloid vessels in PHPV. 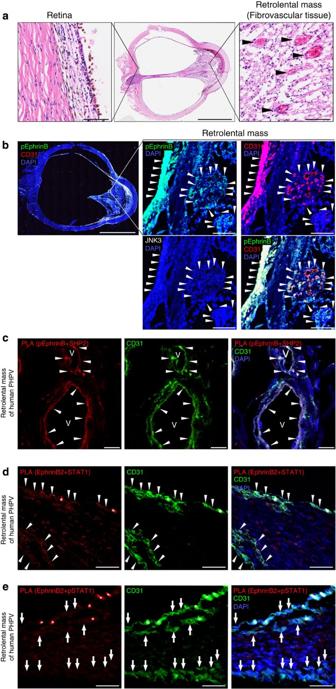Figure 10: Sustained EphrinB2 phosphorylation in endothelial cells within the retrolental mass of PHPV. (a) Retrolental mass and retinal degeneration in PHPV. Cross-section of PHPV eyeball stained with Hematoxylin and Eosin (H&E) (representative of six samples). Center panel: tiled image of the entire eye section showing the characteristic retrolental mass and retinal detachment; scale bar, 5 mm. Left panel: magnified image showing retinal degeneration; scale bar, 100 μm. Right panel: magnified image showing fibrovascular tissue within the retrolental mass; scale bar, 100 μm. (b) Endothelial cells (CD31+) within the PHPV retrolental mass are p-EphrinB+and JNK3−. Staining with anti-p-EphrinB (green), anti-JNK3 (white), anti-CD31 (red) and DAPI (blue). Arrowheads point to CD31+p-EphrinB+JNK3−cells. Scale bars, 1 mm (left panel) and 100 μm (right panels). (c) Proximity co-localization of p-EphrinB and SHP2 in endothelial cells in PHPV retrolental mass. Red: PLA signal from p-EphrinB/SHP2 in section of PHPV retrolental mass; green: CD31 immunostaining; blue: DAPI. V, vessel. Arrowheads point to p-EphrinB+SHP2+cells. Scale bars, 10 μm. (d) PLA showing co-localization of EphrinB2 and STAT1 in endothelial cells from PHPV retrolental mass. Red: PLA signal from EphrinB2/STAT1, green: CD31; blue: DAPI. Asterisk: red blood cell. Arrowheads point to EphrinB2+STAT1+cells. Scale bars, 50 μm. (e) Co-localization of EphrinB2 and p-STAT1 is limited in endothelial cells in PHPV retrolental mass. Red: PLA signal from EphrinB2/p-STAT1, green: CD31; blue: DAPI. Asterisk: red blood cell. Arrows point to EphrinB2+p-STAT1+cells. Scale bars, 50 μm. Figure 10: Sustained EphrinB2 phosphorylation in endothelial cells within the retrolental mass of PHPV. ( a ) Retrolental mass and retinal degeneration in PHPV. Cross-section of PHPV eyeball stained with Hematoxylin and Eosin (H&E) (representative of six samples). Center panel: tiled image of the entire eye section showing the characteristic retrolental mass and retinal detachment; scale bar, 5 mm. Left panel: magnified image showing retinal degeneration; scale bar, 100 μm. Right panel: magnified image showing fibrovascular tissue within the retrolental mass; scale bar, 100 μm. ( b ) Endothelial cells (CD31 + ) within the PHPV retrolental mass are p-EphrinB + and JNK3 − . Staining with anti-p-EphrinB (green), anti-JNK3 (white), anti-CD31 (red) and DAPI (blue). Arrowheads point to CD31 + p-EphrinB + JNK3 − cells. Scale bars, 1 mm (left panel) and 100 μm (right panels). ( c ) Proximity co-localization of p-EphrinB and SHP2 in endothelial cells in PHPV retrolental mass. Red: PLA signal from p-EphrinB/SHP2 in section of PHPV retrolental mass; green: CD31 immunostaining; blue: DAPI. V, vessel. Arrowheads point to p-EphrinB + SHP2 + cells. Scale bars, 10 μm. ( d ) PLA showing co-localization of EphrinB2 and STAT1 in endothelial cells from PHPV retrolental mass. Red: PLA signal from EphrinB2/STAT1, green: CD31; blue: DAPI. Asterisk: red blood cell. Arrowheads point to EphrinB2 + STAT1 + cells. Scale bars, 50 μm. ( e ) Co-localization of EphrinB2 and p-STAT1 is limited in endothelial cells in PHPV retrolental mass. Red: PLA signal from EphrinB2/p-STAT1, green: CD31; blue: DAPI. Asterisk: red blood cell. Arrows point to EphrinB2 + p-STAT1 + cells. Scale bars, 50 μm. Full size image Here we show that EphrinB2 plays a previously unrecognized role as a critical regulator of endothelial cell survival and death controlling vessel pruning once vessels have formed through angiogenesis. EphrinB2 is an essential mediator of angiogenic sprouting that drives tip cell guidance and endothelial cell sprouting by promoting VEGFR2 internalization and signalling [15] , [19] , [22] , [24] . In this context, EphrinB2 relies on PDZ interactions for signalling [15] , [24] . We now discovered that EphrinB2 relies instead on phosphotyrosine-dependent signalling to sustain endothelial cell viability, and find that this function is VEGF/VEGFR2 independent. EphrinB tyrosine phosphorylation is induced by EphB receptors through cell-to-cell interaction [15] and also by FGF2 and Claudins [17] . Since veins, sprouting capillaries [25] , monocyte/macrophages [37] , pericytes [19] and other cells [24] , [38] express EphBs, there is an opportunity for endothelial EphrinB2 activation in vivo . Consistent with this, EphrinB is phosphorylated in the remodelling vasculature of the eye, wounds and tumours [26] . The current results suggest a broader role for EphrinB2 in the vasculature, promoting both vascular sprouting and cell survival through the engagement of distinct signalling pathways. There is growing evidence describing the importance of a dynamic balance between endothelial cell survival, proliferation and cell death during development of the vascular system and in adult angiogenesis [1] , [39] , [40] . The current results show that cessation of EphrinB2 phosphorylation promotes endothelial cell death, suggesting that signals inducing EphrinB dephosphorylation would ensure endothelial cell death when vessel degeneration is needed. Given that cell death is required for vessel pruning, the identification of signals and molecular pathways modulating EphrinB2 phosphorylation in remodelling vessels is an important advance. Endothelial intrinsic signals may involve EphrinB2 recruitment of the phosphatase PTB-BL, which dephosphorylates EphrinB2 (ref. 41 ). Extrinsic signals may originate from endothelium-associated monocytes [37] and pericytes [19] that express EphB4. Pericytes induce vessels pruning contributing to vessel patterning in the eye [29] , a functional role supported by the current results. In contrast to PHPV stemming from hyaloid vessels failing to involute, which is well described [35] , [36] , less is known about pathologies stemming from other vascular structures failing to undergo adaptive pruning since endothelial cell death is rarely detected in tissues, perhaps owing to rapid removal and repair mechanisms [40] . Despite detection difficulties, genetic and biochemical studies have identified several regulators of endothelial cell survival/vascular integrity, including VEGF/VEGFR2 (ref. 7 ), VE (Vascular Endothelial)-cadherin/β-catenin [42] , Netrin-1/UNC5B (ref. 43 ), Birc2 (baculoviral IAP repeat-containing protein-2, also called cIAP1, cellular inhibitor of apoptosis-1; ref. 44 ), Dll4/Notch/Ang2 (ref. 3 ), FGD5 (ref. 10 ) and the sphingosine-1-phosphate receptor S1PR1 (ref. 45 ). JNK3 is expressed in the brain where it mediates neuronal cell death in various models of stress- or trauma-induced neurodegeneration [34] , [46] , [47] and to a lesser degree in all human tissues [34] , [48] . We now discovered that JNK3 induces endothelial cell death, and that JAK2/STAT1 signalling activates JNK3 in endothelial cells. Our results show that hyaloid vessel involution is generally more compromised in mice with JNK3 deficiency than with EphrinB2 phosphotyrosine deficiency, perhaps attributable to compensatory pathways downstream of EphrinB2 signalling. Remarkably, our study links JNK3 deficiency in mice with PHPV in humans attributed to the abnormal persistence of hyaloid vessels [35] , [49] . Previously, deficiencies of angiopoietin-2 (ref. 50 ), p53 (ref. 51 ), Arf [52] , frizzled-5 (ref. 53 ), and Bax and Bak [54] were linked to PHPV development. Whether these deficiencies may be coupled to JNK3 is not clear, but JNK signalling regulates p53 stability [55] and alternative reading frame nuclear translocation [56] . To our knowledge, STAT1 signalling has not been linked to JNK3 regulation, despite the importance of IFNγ-induced STAT1 activation in promoting cell death [57] . Here we show that p-STAT1 induced by IFNγ targets the JNK3 promoter in endothelial cells. Besides potentially contributing to understanding of inflammation-induced vascular damage [58] , this new EphrinB/STAT1/JNK3 pathway suggests that post-angiogenic endothelium in the eye and in other tissues such as tumours, which express tyrosine-p-EphrinB, survives at least in part via repression of JNK3 pro-apoptotic signals. The fully developed, resting vasculature does not usually express active EphrinB, suggesting that other mechanisms must sustain vessel integrity. Many biochemical aspects underlying maturation of nascent vessels are not yet clear [1] . The current results suggest that transition from EphrinB2 phosphotyrosine dependency to independency is a critical step in physiological vessel maturation. Since dephosphorylation of EphrinB2 is expected to lead to accelerated endothelial cell death and vessel regression, the current results disclose novel experimental approaches for inducing vessel pruning. Src family kinases phosphorylate EphrinB2 (refs 41 , 59 ), JAK inhibitors reduce STAT activation and SHP phosphatases inactivate STAT1. Thus, tyrosine kinase inhibitors targeting Src family kinases [60] , SHP inhibitors [61] and JAK inhibitors [62] hold promise for pharmacologically pruning vascular beds that either fail to undergo physiological involution such as hyaloid vessels in PHPV or contribute to disease progression as it is observed in certain cancers types. Mice EphrinB2 WT/WT and EphrinB2 5Y/5Y (ref. 23 ); JNK3 +/− , JNK3 −/− (ref. 34 ; all C57BL/6 genetic background) and control C57BL/6 (Jackson Laboratories) mice were used in compliance with protocols approved by the National Cancer Institute Institutional Animal Care and Use Committee. Cells, gene silencing and expression HUVEC (derived from umbilical vein by collagenase (type II) dissociation) and HDMEC (Clonetics, no. CC-2543) were cultured in EGM-2MV BulletKit (Clonetics, no. CC-3156 and CC-4176); human mesenchymal (Lonza, no. PT-2501) stem cells (MSCs) were cultured in MSC growth medium (Lonza, no. PT-3001) and 293 T cells (ATCC, no. CRL-3216) were cultured in Dulbecco’s modified Eagle’s medium (Gibco Life Technologies, no. 110965-092) with 10% fetal bovine serum (FBS; Sigma-Aldrich, no. F2442-500ML; refs 26 , 63 ). Co-culture experiments with HUVEC and MSC were performed by adding a mixture of these cell populations (HUVEC 4 × 10 4 cells and MSC 2 × 10 4 cells in 500 μl HUVEC culture medium) onto 24-well plates pre-coated with Matrigel (200 μl; Corning, no. 356237) and incubating 18 h at 37 °C (ref. 26 ). For EphrinB2 silencing, we used third-generation lentiviral vectors ([Vsv-g]-pseudotype HIV-1-based; shRNA) [26] . For overexpression of EphrinB2, we generated lentiviral vectors by subcloning EYFP-HA-EphrinB2-WT, EYFP-HA-EphrinB2-5Y and EYFP plasmids [23] , [64] (gifts of T. Makinen, Cancer Research UK) into the 277.pCCLsin.PPT.hPGK.GFP.pre transfer vector [65] (gift of A. Follenzi, Albert Einstein College of Medicine, NY). The EYFP-EphrinB2-5Y vector was derived from EYFP-EphrinB2-WT plasmid [26] . To generate lentiviral particles, 277.pCCLsin.PPT.hPGK.GFP.pre transfer vector was co-transfected with pRSV-Rev, pMDLg/pRRE, pLP/VSVG into 293 T cells. ON-TARGETplus short interfering RNA (Dharmacon, no. L-003543-00-0005) and Risc-free control short interfering RNA (Dharmacon, no. D-001600-01-05) were used for silencing STAT1 expression [26] . Expression vectors for JAK2-HA, DN-JAK2-HA (gifts of I. Daar, NCI, NIH), STAT1-GFP (Addgene, no. 11987) and JNK3 mCherry (GeneCopoeia, EX-A1150-M55) were transfected into HUVEC and HDMEC [30] . MISSION shRNA was used for silencing JNK3 expression (Sigma-Aldrich, no. SHCLND-NM_002753). Quantitative PCR was used to measure mRNAs [26] , [63] . IP and immunoblotting HUVEC were cultured for 6 h in Medium 199 (Life Technologies, no. 11150-059) containing 20% FBS, 10 ng ml −1 VEGF (R&D Systems, no. 293-VE-010), 10 ng ml −1 FGF2 (R&D Systems, no. 233-FB-025), 10 ng ml −1 IGF-1 (R&D Systems, no. 291-G1-200), 10 ng ml −1 EGF (R&D Systems, no. 236-EG-200), 25 μg ml −1 heparin (Sigma-Aldrich, no. H3149), 100 μM sodium orthovanadate (Sigma-Aldrich, no. S6508), 50 μg ml −1 ascorbic acid (Sigma-Aldrich, no. A4544), 2 mM L-glutamine (Gibco Invitrogen, no. 25030-081) and 100 U ml −1 penicillin per 100 μg ml −1 streptomycin (Gibco Invitrogen, no. 15140-122). Cells were collected with 0.5% NP-40 lysis buffer (25 mM Tris-HCl (pH 7.4) 137 mM NaCl, 3 mM KCl, 0.5% IGEPAL CA-630, 0.1 mM CaCl 2 , 0.1 mM MgCl 2 , 1 mM sodium orthovanadate, 20 mM sodium fluoride, 25 mM sodium pyrophosphate, 10% glycerol, proteinase inhibitor cocktail and EDTA-free (Roche, no. 11836170001). Cell lysate supernatant was incubated with rabbit anti-EphrinB (8 μg ml −1 , Santa Cruz Biotechnology, no. sc-910) or normal rabbit IgG (8 μg ml −1 , Santa Cruz Biotechnology, no. sc-2027) overnight at 4 °C. Immunoprecipitates and IP input were analysed by SDS-PAGE and immunoblotting. The following primary antibodies were used for immunoblotting: rabbit monoclonal or polyclonal IgG antibodies to SHP2 (no. 3397; 1:1,000), p-VEGFR2 (Tyr 1175 ) (no. 2478; 1:1,000); VEGFR2 (no. 2479; 1:1,000); p-Erk (Thr 202 /Tyr 204 ) (no. 4370; 1:2,000); Erk (p44/p42) (no. 9102; 1:1,000); p-EphrinB (Tyr 324/ Tyr 329 ) (no. 3481; 1:1,000); cleaved poly (ADP-ribose) polymerase (Asp 214 ) (no. 5625; 1:1,000); JNK3 (no. 2305; 1:1,000); JAK2 (no. 3230; 1:1,000); p-JAK2 (Tyr 1007/1008 ) (no. 3776; 1:1,000); STAT1 (no. 9175; 1:1,000); p-STAT1 (Tyr 701 ) (no. 9167; 1:1,000); p-STAT3 (Tyr 705 ) (no. 9145; 1:2,000) (all obtained from Cell Signaling Technologies); goat anti-SHP2 (Abcam, no. Ab110194; 1:250); rabbit anti-JNK3 (Novus Biologicals, no. NBP!-19542; 1:2,000) and goat anti-actin (Santa Cruz Biotechnology, no. sc-1616; 1:5000). Secondary antibodies HRP-conjugated donkey anti-rabbit IgG (no. NA934V; 1:10,000) or HRP-conjugated donkey anti-goat IgG-Fc (no. NA931V; 1:10,000) (both from GE Healthcare Life Sciences ) were visualized by HRP chemioluminescent substrate (Millipore no. RPN216) or Super Signal West Fento Maximum Sensitivity Substrate (Thermo-Scientific, no. 34095) Membranes were stripped and restained. Secondary antibodies for IP detection were clean-blot IP Detection reagent (Thermo-Scientific no. 212320; 1:1,000). Full-size images of western blot scans are presented in Supplementary Figs 9–13 . Chromatin IP Cells were fixed with fresh 1% formaldehyde (final concentration) in Medium 199 for 10 min at room temperature. Fragmented chromatin was prepared using SimpleChIP Enzymatic Chromatin IP kit (Cell Signaling Technologies, no. 9003). Chromatin IP was performed with rabbit anti-p-STAT1 (Tyr701; Cell Signaling Technologies, no. 9167; 1:80), rabbit anti-histone H3 (a technical positive control, Cell Signaling Technologies, no. 4620; 1:40) and normal rabbit IgG (a negative control, Cell Signaling Technologies, no. 2729, 2.5 μg ml −1 ). After reverse crosslinking and DNA purification, immunoprecipitated DNA was quantified by real-time PCR using SYBR Green (Roche, no. 04673484001) with primers for a STAT1 binding site in the JNK3 promoter (forward primer 5′-GGTTTCCAGGCAGTGAAAGA-3′, reverse primer 5′-GAATTGAGGGGTGAGGACAA-3′), IFN regulatory factor 1 (forward primer 5′-AAGAGGGAAGAAGGCAGAGG-3′, reverse primer 5′-GGGAATCCCGCTAAGTGTTT-3′) and RPL30 exon 3 (Cell Signaling Technologies, no. 7014). Fold enrichment was calculated based on Ct value of IgG control using the comparative Ct method. JNK in vitro kinase assay JNK in vitro kinase assay was performed using JNK kinase assay kit (Cell Signaling Technologies, no. 8794) according to the manufacturer’s protocol. Briefly, HUVEC were cultured for 0, 1, 3, 6, 7, 9 and 10 h in Medium 199 (Life Technologies, no. 11150-059) containing 25 μg ml −1 heparin (Sigma-Aldrich, no. H3149), 50 μg ml −1 ascorbic acid (Sigma-Aldrich, no. A4544), 2 mM L-glutamine (Gibco Invitrogen, no. 25030-081), 100 U ml −1 penicillin and 100 μg ml −1 streptomycin (Gibco Invitrogen no. 15140-122). Phosphorylated JNKs were immunoprecipitated with rabbit anti-phospho-SAPK/JNK (Thr183/Tyr185, Cell Signaling Technologies, no. 4306; 1:20). The immunoprecipitates were reacted with recombinant cJUN fusion protein (Cell Signaling Technologies, no. 6093). After the reaction, the immunoprecipitates and the recombinant cJUN protein were analysed by SDS-PAGE and western blotting with rabbit anti-phospho-cJUN (pS63, Epitomics, no. 527-1; 1:1,000), rabbit anti-cJUN (Epitomics, no. 1254-1; 1:1,000), mouse anti-JNK1 (Cell Signaling Technologies, no. 3708; 1:1,000), rabbit anti-JNK2 (Cell Signaling Technologies, no. 4672; 1:1,000) and rabbit anti-JNK3 (Cell Signaling Technologies, no. 2305; 1:1,000). Reporter assays A transfection-ready Gaussia luciferase (Gluc)-ON dual-reporter vector system pEZX-PG04 that uses GLuc as the promoter reporter upstream JNK3 promoter sequences and SEAP (secreted alkaline phosphatase) as the internal control for normalization (GeneCopoeia, no. HPRM23021-PG04) was included in co-transfection mixtures with expression plasmids for JAK2 (a gift of I. Daar, NCI, NIH) and STAT1 (Addgene, ID no. 12301) or DN-JAK2 (A gift of I. Daar, NCI, NIH) and STAT1 alone, with EphrinB2WT or with EphrinB2-5Y. Supernatants (obtained 48–72 h after HEK293T transfection) were monitored for GLuc and SEAP activities, using Secrete-Pair Dual Luminescence Assay Kit (GeneCopeia, no. SPDA-D010). Optima luminometer was used to inject 100 μl of GLuc and SEAP Assay Kit substrate, and light emission (in relative light units) was measured according to manufacturer’s instructions. Flow cytometry and proliferation Cell viability/death was measured by flow cytometry after 20 min cell incubation with Hoechst 33342 (Life Technologies, no. H3570; 1 μg ml −1 ) and propidium iodide (Life Technologies, P3566; 3 μM); levels of p-STAT1 and p-STAT3 were measured by flow cytometry after cell fixation (4% paraformaldehyde (PFA), 10 min at room temperature), permeabilization (90% methanol, 30 min at 4 °C) and wash (twice in cold PBS, 0.5% bovine serum albumin, protease and phosphatase inhibitors) by immunostaining with phospho-STAT1 (Tyr701) rabbit mAb (Cell Signaling Technologies, no. 9167; 1:200) or p-STAT3 (Tyr 705 ) rabbit mAb (Cell Signaling Technologies, no. 9145; 1:200); bound antibody was detected with Alexa Fluor 647-conjugated anti-rabbit IgG (Life Technologies, no. A-20991; 1:500; refs 26 , 63 ). Endothelial cell proliferation was measured by IncuCyte imaging [63] . EphB4-Fc Chimera (R&D Systems, no. 446-B4-200; 10 μg ml −1 ) and control IgG-Fc (R&D Systems, no. 110-HG-100; 10 μg ml −1 ) was used to activate EphrinB2 (ref. 24 ). Immunofluorescence Endothelial cells grown on gelatin-coated glass chamber slides were fixed in 4% PFA. Mouse eye balls were fixed with 2% or 4% PFA overnight or 4 h at 4 °C, and the sclera was removed under stereomicroscopy (Stemi SV11, Carl Zeiss). Hyaloid vessels and retinas were prepared from the retinal cup [63] that was blocked and permeabilized with blocking buffer (PBS containing 1% Triton X-100, 10% FBS, 10 mM glycine, 0.1 mM CaCl 2 and 0.1 mM MgCl 2 , or PBS containing 0.1% Tween20 and bovine serum) for 1 h. Paraffin-embedded human PHPV specimens (from anonymized excess tissue not required for diagnosis acquired with approval of Johns Hopkins IRB: Institutional Review Board; protocol: ‘Pathological analysis of ocular trauma and other non-neoplastic eye diseases’) were sectioned with a microtome (Leica RM2155, Leica Biosystems) at 10 μm. The sections were deparaffinized with xylene and ethanol, and then re-fixed with 4% PFA on a glass slide TRUBOND 360 (Tru Scientific, no. 5079W) for 20 min at room temperature. The sections were treated with Uni-Trive solution (Inovex Bioscience, no. NB325) at 70 °C for 30 min. After blocking, retinal cup and a section of PHPV specimens were incubated (overnight, 4 °C) with rabbit anti-collagen IV (1:100, Abd Serotec, no. 2150-1470), rabbit anti-phospho EphrinB (1:100, Cell Signaling Technologies, no. 3481), rabbit anti-cleaved caspase-3 (1:300, Cell Signaling Technologies, no. 9579), rabbit anti-JNK3 (1:50, Novus Biologicals, no. NBP1-19542), rat anti-mouse F4/80 (1:50, Abd Serotech, no. MCA497GA), rabbit anti-mouse NG2 (1:200, Millipore, no. AB5320) or rabbit anti-mouse Ki67 (D3B5; 1:100, Cell Signaling Technologies, no. 9129) plus biotinylated isolectin B4 (1:100, Life Technologies, no. I21414) or rat anti-mouse CD31/PECAM (1:100, Dianova, no. DIA-310 or BD Pharmingen, no. 553370). The retina was further incubated for 1 h at 4 °C with Alexa Flour 488- (no. A-21206), 594- (no. A-11056) or 647- (no. A-21244) conjugated anti-rabbit IgG (1:2,000, Life Technologies) or Alexa Flour 488- (no. A-11055), 594- (no. A-11056) or 647- (no. A-21447) conjugated anti-goat IgG (1:2,000, Life Technologies) plus Alexa Fluor 488- (no. S-11223) or 647- (no. S-32357) conjugated streptavidin (1:200, Life Technologies) or Alexa Flour 647-conjugated donkey anti-rat IgG (1:400, Life Technologies, no. A-21247). For retinal staining, signal was visualized using biotinylated anti-rabbit IgG (1:200, Vector Laboratories, no. BA-1000) plus Alexa Flour 594-conjugated streptavidin (1:200, Life Technologies). For JNK3 (Novus Biologicals, no. NBP1-19542; 1:400) and p-EphrinB (Cell Signaling Technologies, no. 3481, 1:100) double staining, anti-JNK3 was visualized with AlexaFluor 594-labelled anti-rabbit IgG (H+L, 1:200, Life Technologies, no. A-21207). After blocking with normal rabbit IgG (Vector Laboratories, no. S5000), p-EphrinB was visualized with Zenon-labelled (Labelling kit from Life Technologies no. Z-25302) AlexaFluor 488-Rabbit anti-p-EphrinB (1:100, Cell Signaling Technologies, no. 3481). Images were obtained with Carl Zeiss LSM 710NLO (Carl Zeiss) or LSM 780 (Carl Zeiss) microscopes using ZEN software (Carl Zeiss). Image quantification The number of vessel branch points ( Figs 1b and 4b ) and joints ( Fig. 5f ) was counted with ImageJ software (NIH) [26] . To measure branch points of hyaloid vessels ( Supplementary Fig. 5c ), we used four images each from four whole hyaloid vessels at p4, p5 and p7 stained with IB4. The image of the whole hyaloid vessels was divided in 10 regions based on relative distance from the central optic nerve to the periphery using ImageJ. The area was measured by ImageJ and converted pixels into mm 2 . The number of branch points in each region was measured by ImageJ and was divided by the area providing the average number of branch points of hyaloid vessels per mm 2 in each region. To measure collagen IV + /CD31 − sleeves in hyaloid and retinal vessels ( Figs 1e and 4b ), we used four images each from four whole hyaloid vessels at p4 stained with anti-collagen IV and anti-CD31. In Figs 4d four fields of retina were used for this analysis. We used ImageJ with ‘Segmented line tool and ROI manager’ to measure the length of collagen IV + CD31 − sleeves. The average length of collagen IV + CD31 − sleeves in whole hyaloid vessels is shown. In Fig. 4d , the length of collagen IV + CD31 − sleeves was divided by the length of CD31 + vessels and the average ratio was shown. To measure Ki67 + CD31 − cells in hyaloid and retinal vessels ( Figs 1g and 4f ), we counted by ImageJ using ‘Analyze Particle tools’ the nuclei of Ki67 + CD31 + cells and the total number of vascular CD31 + cells in hyaloid and retinal vessels. The percentage of Ki67 + CD31 + cells in CD31 + vascular cells was calculated and the average ratios were shown. To count the number of red blood cells in hyaloid vessels ( Fig. 2b,c ), hyaloid vessels were stained with biotinylated IB4, and then stained with AlexaFluor 546-labelled streptavidin. To enhance autofluorescence of red blood cells in hyaloid vessels, flattened hyaloid vessels were fixed with 1% glutaraldehyde/3.8% PFA in PBS for 20 min at room temperature. Images were obtained with Carl Zeiss LSM 780 (Carl Zeiss) microscope using ZEN software (Carl Zeiss). Excitation was induced with argon laser (488 nm) and HeNe laser (561 nm), and emission was detected for green fluorescence at 495–535 nm and for red fluorescence at 565–600 nm. Green and red autofluorescence-positive cells were counted as red blood cells using ImageJ software (NIH). The length of hyaloid vessels was measured by ImageJ software. The number of red blood cells was divided by the length of hyaloid vessels. To measure vessel perfusion with fluorescein isothiocyanate (FITC)-dextran ( Fig. 2f ), 40 μl PBS containing FITC-dextran (2,000,000 mol wt, Sigma-Aldrich, no. FD2000S; 50 mg ml −1 ) and poly-L-lysine (300 kDa, Sigma, no. P-1524; 10 mg ml −1 ) were injected retro-orbitally into p4 littermate EphrinB2 WT/WT and EphrinB2 5Y/5Y mice. After 5 min, the pups were euthanized, eyes collected and fixed with 4% PFA overnight at 4 °C. Sclera was removed under a stereomicroscope. Hyaloid vessels were prepared, stained with IB4 and flattened with 4% low-melting temperature agarose in DPBS: Dulbecco's PBS [63] . Images were acquired with a Zeiss LSM780 microscope (Carl Zeiss). The total intensity of FITC-dextran in whole hyaloid vessels and the total length of whole hyaloid vessels were measured by ImageJ. The total intensity of FITC-dextran was divided by the length of hyaloid vessels. The results are shown as the average intensity of FITC-dextran per mm hyaloid vessel. To measure cleaved caspase-3 intensity in endothelial cells and macrophages ( Fig. 3c,d ), hyaloid vessels at p4 were stained with anti-cleaved caspase-3, IB4 and 4,6-diamidino-2-phenylindole (DAPI). Images were acquired with a Zeiss LSM780 microscope. Region of interest (ROI) setting for macrophages and endothelial cells was set by ImageJ Using the ROI, total intensity was divided by the area of individual cells. Mean intensity of cleaved caspase-3 in individual cells was plotted in Fig. 3c,d . Individual dots are representative of single cells. To count NG2 + pericytes ( Fig. 3g ) and F4/80 + macrophages, hyaloid vessels at p4 were stained with anti-NG2 or anti-F4/80, IB4 and DAPI. Images were acquired by Zeiss LSM780 (Carl Zeiss). ROI setting for NG2 + pericytes, NG2 − IB4 + vascular endothelial cells, F4/80 + macrophages and F4/80 − IB4 + vascular endothelial cells were set by ImageJ. The number of NG2 + pericytes, NG2 − IB4 + vascular endothelial cells, F4/80 + macrophages and F4/80 − IB4 + vascular endothelial cells were counted using the ROI settings. The number of NG2 + pericytes was normalized by the number of NG2 − IB4 + vascular endothelial cells. The average number of NG2 + pericytes/100 NG2 − IB4 + vascular endothelial cells and F4/80 + cells/100 F4/80 − IB4 + vascular endothelial cells is shown in Fig. 3g and Supplementary Fig. 2 , respectively. For quantification of JNK3 and p-EphrinB fluorescence intensity in individual endothelial cells ( Fig. 7i,j ), ROIs were generated by ImageJ software (NIH) based on DAPI staining of hyaloid vessels. The ROIs were applied to images of hyaloid vessels stained for JNK3 and p-EphrinB. After applying the ROIs, total intensity of JNK3 and p-EphrinB, and area in each ROI were measured by ImageJ. Mean intensity of JNK3 and p-EphrinB in each ROI was calculated by dividing the total intensity of JNK3 and p-EphrinB by the area of each ROI. In Fig. 7i , the mean intensities of JNK3 and p-EphrinB staining in each ROI are shown as a dot plot. To measure the fluorescence intensity of JNK3 and p-EphrinB in each region of hyaloid vessels ( Fig. 7k ), an image of hyaloid vessels was divided into 10 regions based on relative distance from the centre (optic nerve) to the periphery using ImageJ. Fluorescence intensity of JNK3 and p-EphrinB in each region of hyaloid vessels was measured by ImageJ, and was subsequently normalized by DAPI fluorescence intensity in each region to adjust for different cell number in each region (there is a cell number gradient from the centre to the periphery of hyaloid vessels). For three-dimensional reconstitution and surface rendering of sprouting hyaloid vessels in retina ( Supplementary Fig. 7 ), Z stack images were acquired by Zeiss LSM780 from 0.5 μm thickness/layers and processed using Imaris software (Bitplane Scientific software). Proximity ligation assay PLA was used to visualize proximity co-localization (<40 nm) of EphrinB2+JAK2, EphrinB2+STAT1 and EphrinB2+SHP2 in HUVEC and hyaloid vessels using Duolink Detection kit (Olink Bioscience, Uppsala, Sweden). The cells were fixed with 4% PFA for 20 min at room temperature. Flattened mouse hyaloid vessels were embedded in 4% hydrogel solution (4% acrylamide, 0.05% bis-acrylamide and 0.25% VA044 photoinitiator (Wako, no. VA044), and 4% PFA in PBS), and then incubated for 3 h at 37 °C. Paraffin-embedded sections of human PHPV were deparaffinized with xylene and ethanol, and then re-fixed with 4% PFA for 20 min at room temperature. Mouse hyaloid vessels and sections of human PHPV were treated with Uni-Trieve solution (Innovex Biosciences, no. NB325) at 70 °C for 30 min. After blocking, cells, mouse hyaloid vessels and sections of human PHPV were incubated overnight at 4 °C with rabbit anti-JNK3 (1:50, Novus Biologicals, no. NBP1-19542)+mouse anti-JNK3 (1:500, Abnova, no H00005602-M01), rabbit anti-p-EphrinB (1:200, Cell Signaling Technologies, no. 3481)+goat anti-SHP2 (1:133, Abcam, no. ab110194), rabbit anti-EphrinB2 (1:100, Abcam, no. ab131536)+mouse anti-STAT1 (1:20, Abcam, no. ab2415), rabbit anti-EphrinB2 (1:100, Abcam, no. ab131536)+mouse anti-STAT1 (1:100, Abcam, no. ab2415), goat anti-EphrinB2 (1:50, R&D Systems, no. AF496)+rabbit anti-JAK2 (1:100, Cell Signaling, no. 3230) and goat anti-EphrinB2 (1:50, R&D Systems, no. AF496)+rabbit anti-STAT1 (1:100, Cell Signaling, no. 9175). After washing, cells, hyaloid vessels and sections were incubated with secondary antibodies with PLA probes (MINUS probe-conjugated anti-rabbit IgG+PLUS probe-conjugated anti-mouse IgG for JNK3, EphrinB2+STAT1 and EphrinB2+-STAT1 detection; PLUS probe-conjugated anti-goat IgG+MINUS probe-conjugated anti-rabbit IgG for detection of EphrinB2+JAK2, EphrinB2+STAT1 and EphrinB2+SHP2; Olink Bioscience, Uppsala, Sweden). Circularization and ligation of the oligonucleotides in the probes was followed by an amplification step. A complementary fluorescent-labelled probe was used to detect the product of rolling circle amplification. The cells and the sections of human PHPV were stained with AlexaFluor 488-Zenon-labelled mouse anti-human CD31 (Covance/Biolegend, no. SIG-3632). Slides were mounted with Duolink II Mounting Medium containing DAPI. Images were obtained with Carl Zeiss LSM 710NLO (Carl Zeiss) or LSM 780 (Carl Zeiss) using ZEN software (Carl Zeiss). In HUVEC, the number of PLA dots was counted using ImageJ software (NIH). Quantifications are given as mean±s.d. Hyaloid vessels were divided into 10 regions based on distance from centre (optic nerve) to periphery. Total intensity of PLA, total intensity of DAPI staining and total area was measured by ImageJ software in the each region. Total intensity of PLA signal in each region was divided by area (=total intensity per mm 2 ). Hyaloid vessel density differs in different regions. Total intensity of PLA signal per mm 2 was normalized by total intensity of DAPI staining. Proximity extension assay We applied PEA [66] to detect protein complexes in lysates of hyaloid vessels. Lysates were prepared from hyaloid vessels of EphrinB2 WT/WT and EphrinB2 5Y/5Y mice at p5 with lysis buffer (25 mM Tris-HCl (pH 7.4) 137 mM NaCl, 3 mM KCl, 0.5% IGEPAL CA-630, 1 mM sodium orthovanadate, 20 mM sodium fluoride, 25 mM sodium pyrophosphate, 50% glycerol and proteinase inhibitor cocktail). Lysates are stored at −20 °C until use. Protein concentration in the lysate was adjusted to 0.5 mg ml −1 . Antibodies were labelled with Proseek Probemaker (Olink Bioscience); anti-EphrinB2 rabbit monoclonal antibody (Abcam, no. 150411) was labelled with oligo DNA probe A; anti-SHP2 rabbit monoclonal antibody (Cell Signaling Technologies, no. 3397), anti-JAK2 rabbit monoclonal antibody (Cell Signaling Technologies, no. 3230) and anti-STAT1 rabbit polyclonal antibody (Cell Signaling Technologies, no. 9172) were labelled with oligo DNA probe B according to the manufacturer’s protocol; PEA was performed using Proseek Assay Development Kit (Olink Bioscience) according to the manufacturer’s protocol. Briefly, probe A- and probe B-labelled antibodies were diluted to 65 pM with assay solution, and then mixed with the lysate. After incubation, the region annealed by probe A and probe B (based on proximity co-localization of the proteins in the lysate) was extended by DNA polymerase. The extended DNA product was quantified by real-time PCR with a specific TaqMan probe. The lysis buffer without hyaloid vessels was used as a negative control for PEA. The negative control was used as background. Fold increase of each complex was calculated based on Ct value of the negative control by the comparative Ct method. Input of SHP2, JAK2 and STAT1 content was measured by western blotting using the same lysate used in the PEA. Statistical analysis The results are presented as mean±s.d. The statistical significance of differences between two groups was calculated using two-tailed Student t -test. The results are provided as P values, where P <0.05 is considered significant. How to cite this article: Salvucci, O. et al . EphrinB2 controls vessel pruning through STAT1-JNK3 signalling. Nat. Commun . 6:6576 doi: 10.1038/ncomms7576 (2015).